Retrospective evaluation of whole exome and genome mutation calls in 746 cancer samples 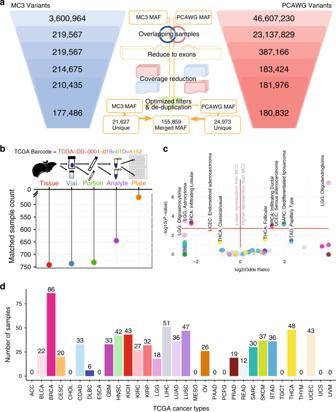Fig. 1: Workflow and sample inclusion statistics. aA workflow diagram illustrates the number of mutations present during each step (gradient) of the filtering processes for MC3 (left, blue) and PCAWG (right, red). A brief description of each step of the intersection process is shown in between.bTCGA barcodes and aliquot IDs were used to match somatic sequencing. The exact match of these IDs is shown for various collection aliquots from tissue to plate.cA volcano plot highlights cancer subtype discrepancy between each PCAWG and MC3 with −log10(p-value) on they-axis and log2(odds ratio) on thex-axis (Fisher’s exact test). The horizontal red bar indicates a significant threshold after multiple testing correction. Positive values indicate an over-representation of a cancer subtype in PCAWG, while negative values indicate an under-representation of a cancer subtype in PCAWG compared to MC3-separated by a vertical red bar.dSample counts for each cancer type are shown in a bar chart. The colors coordinate with panelc. The Cancer Genome Atlas (TCGA) and International Cancer Genome Consortium (ICGC) curated consensus somatic mutation calls using whole exome sequencing (WES) and whole genome sequencing (WGS), respectively. Here, as part of the ICGC/TCGA Pan-Cancer Analysis of Whole Genomes (PCAWG) Consortium, which aggregated whole genome sequencing data from 2,658 cancers across 38 tumour types, we compare WES and WGS side-by-side from 746 TCGA samples, finding that ~80% of mutations overlap in covered exonic regions. We estimate that low variant allele fraction (VAF < 15%) and clonal heterogeneity contribute up to 68% of private WGS mutations and 71% of private WES mutations. We observe that ~30% of private WGS mutations trace to mutations identified by a single variant caller in WES consensus efforts. WGS captures both ~50% more variation in exonic regions and un-observed mutations in loci with variable GC-content. Together, our analysis highlights technological divergences between two reproducible somatic variant detection efforts. Complementary efforts of The Cancer Genome Atlas (TCGA) and the International Cancer Genome Consortium (ICGC) have recently produced two of the highest quality and most elaborate and reproducible somatic variant call sets from exome and whole genome-level data in cancer genomics, respectively. The motivation for these efforts stems from the notion that “scientific crowd sourcing” and combining mutation callers can provide very strong results. These two efforts produced variant calls from 10 different callers, namely Radia [1] , Varscan [2] , MuSE [3] , MuTect [4] , Pindel [5] , [6] , Indelocator [7] , SomaticSniper [8] for WES and MuSE, Broad-Pipeline (anchored by MuTect), Sanger-pipeline, German Cancer Research Center pipeline (DKFZ), and SMuFin [9] , for WGS. Briefly, the PCAWG Consortium aggregated whole genome sequencing data from 2658 cancers across 38 tumor types generated by the ICGC and TCGA projects. These sequencing data were re-analyzed with standardized, high-accuracy pipelines to align to the human genome (reference build hs37d5) and identify germline variants and somatically acquired mutations [10] . Of the 885 TCGA samples in ICGC, 746 were included in the latest exome call set produced by both the Multi-Center Mutation Calling in Multiple Cancers (MC3) effort and the Pan-Cancer Analysis of Whole Genomes (PCAWG) Consortium set. These 746 samples represent a critical benchmark for high-level analysis of similarities and differences between exome and genome somatic variant detection methods. Reproducibility of mutations identified by both whole exome capture sequencing and whole genome sequencing (WGS) techniques remains an important issue, not only for the scientific use of large, established data sets, but for data designs of future research projects. Previous work analyzing exome capture effects on sequence read quality has shown that GC-content bias is the major source of variation in coverage [11] . A performance comparison across exome-captured platforms demonstrated that for most technologies, both high and low GC-content result in reduced coverage in read depth [12] . Belkadi et al. compared mutation calls between WGS and WES, observing that ~3% of coding variants with high quality were only detected in WGS, and WGS also had a more uniform distribution of coverage depth, genotype quality, and minor read ratio [13] . Furthermore, due to the relatively high error rate per read in next-generation sequencing [14] , the detectability of mutations with low variant allele fractions (VAFs) is limited by background noise. Despite these studies’ nuanced preference towards WGS, others contend that WES will remain a better choice until costs of WGS fall [15] . The decision to sequence exomes or whole genomes is further confounded as more recent publications in oncology select either WGS [16] , [17] , [18] , [19] , [20] or WES [21] , [22] , [23] , [24] . Recognizing the unresolved nature of this issue, Schwarze et al. have called for more comprehensive studies comparing the WES and WGS studies, especially as this issue has important ramifications for the clinic [25] . Our analysis provides confidence that mutation calls within the captured exonic regions of these two data sets are largely consistent. We highlight common sample, cohort, and caller-specific challenges in cancer variant detection from the TCGA and ICGC efforts. We show that variants that are most confidently called in one database i.e., called by multiple callers, are very likely to be called in the other. We assess how reproducibility impacts higher-level mutation signature analysis and illustrate the need for caution in assessing performance that can only be identified by the overlap of these two data sets. Finally, we explore the capacity of WGS to detect recurrent non-coding mutations captured by whole exome sequencing. Data and workflow We used publicly available data from the MC3 and PCAWG repositories, consisting of ~3.6 M and ~47 M variants, respectively (Fig. 1a ). 746 samples were sequenced by both WES and WGS, comprising various aliquots and portions of the same tumor (Supplementary Data 1 , Fig. 1b ). Effects of these differences are discussed below for preliminary results, but we ultimately used the entire set of 746 samples in the variant overlap analysis, since the effects of tumor partitioning did not play a significant role (Supplementary Fig. 1 ). By restricting the public data sets to overlapping samples, we reduced the total corpus to ~220 K (6.1%) and ~23 M (49.6%) mutations for exome and whole genome, respectively. It is notable that there is an enrichment of variants in hypermutated samples from COAD, HNSC, LUAD, and STAD in the PCAWG set used in this study (Supplementary Fig. 2 ). To begin building a comparable set of mutations between these two studies, we further restricted the whole genome data set to exon regions provided by the MC3 analysis working group. This reduced the WGS data set to 1.6% of its original size, within range of total exome material estimations [26] (Fig. 1a ). The next step involved removing poorly-covered variants potentially caused by technical anomalies by limiting mutations to those captured in coverage files (distributed as.wig files). A reciprocal coverage strategy was used, meaning PCAWG mutations were restricted to covered genomic regions in MC3 and vice versa, thereby maintaining a complementary set of callable genomic regions. Removal of mutations in uncovered regions reduced the remaining PCAWG data set by approximately one-half, from 387,166 to 183,424 mutations. We also identified 4241 MC3 and 2219 PCAWG mutations that were present in the respective MAF but were not marked as covered in the coverage files provided by a single group. This suggests that different tools consider different minimum coverage strategies. These mutations reflect 2.0% and 1.2%, respectively, of the total mutation discrepancy and were removed because some callers had limited capacity to identify mutations in poorly-covered regions (see “Methods” section). Finally, filter flags provided by MC3 were used to assess somatic mutation filtering strategies. At this stage, we performed filter optimization to comprehensively evaluate all possible combinations of MC3 filters (Supplementary Fig. 3a ). Ultimately, we decided to only remove OxoG labeled artifacts and duplicated events produced by these filters (see “Methods” section, Supplementary Data 2 ). Since each stage of this filtering workflow resulted in many alternative decisions and outcomes, we built MAFit, a web-based graphical user interface that allows users to easily customize comparisons of merged mutations ( https://mbailey.shinyapps.io/MAFit/ ). A MC3 filter assessment also shows that many variants with filter flags in MC3 are present in the PCAWG variant call set, suggesting a need for improved filtering strategies (Supplementary Fig. 3b ). Fig. 1: Workflow and sample inclusion statistics. a A workflow diagram illustrates the number of mutations present during each step (gradient) of the filtering processes for MC3 (left, blue) and PCAWG (right, red). A brief description of each step of the intersection process is shown in between. b TCGA barcodes and aliquot IDs were used to match somatic sequencing. The exact match of these IDs is shown for various collection aliquots from tissue to plate. c A volcano plot highlights cancer subtype discrepancy between each PCAWG and MC3 with −log10( p -value) on the y -axis and log2(odds ratio) on the x -axis (Fisher’s exact test). The horizontal red bar indicates a significant threshold after multiple testing correction. Positive values indicate an over-representation of a cancer subtype in PCAWG, while negative values indicate an under-representation of a cancer subtype in PCAWG compared to MC3-separated by a vertical red bar. d Sample counts for each cancer type are shown in a bar chart. The colors coordinate with panel c . Full size image TCGA samples comprise a sizable fraction of the PCAWG sample pool (~30%, Supplementary Data 1 ) Additional WGS sequencing from TCGA allowed for mutation validation [27] and insights into non-coding mutations, such as in TET2 . However, this selection process could have potentially influenced our basic comparison of exome-sequenced samples and genome-sequenced samples in two fundamental ways. First, vagaries of tumor extraction and tissue storage protocols may have resulted in many different portions of a tumor being stored, introducing the possibility that different subclones of the same tumor could be present. These could have very different genetic makeups. This information was captured in different substrings of the TCGA identification barcode (see “Methods” section). From the 746 TCGA barcodes, we found that 64% (477) could be traced to the same well of a microtiter plate (Fig. 1b ). After correcting for cancer type, we modeled both the impact of matching barcode identifiers between MC3 and PCAWG and variant concordance, finding that differing barcodes did not have an appreciable impact. This result was seen for all samples, even when excluding the hypermutator (Fig. 1 ). Second, each AWG was able to independently select samples for WGS, which, while not affecting mutation calling, does raise potential biases when comparing PCAWG results to TCGA exome cohort data. An enrichment analysis was performed to identify which tumor subtypes may have been preferentially selected for different cancer types. We found that four tumor subtypes were enriched in the PCAWG effort from TCGA samples: infiltrating ductal breast cancer, endometrial serous adenocarcinoma, differentiated liposarcoma, and low grade oligodendroglioma (FDR < 0.05, Fig. 1c , Supplementary Data 3 , and see “Methods” section). Final tumor sample counts for each cancer type are shown in Fig. 1d . Landscape of mutational overlap between WGS and WES calls Limiting our analysis to coding regions with sufficient coverage yielded a total of 202,459 variants (155,859 matched, 21,627 unique MC3 variants, and 24,973 unique PCAWG mutations), with 76.7% in concordance between MC3 and PCAWG and 10.7% and 12.3% being unique in MC3 and PCAWG, respectively (Fig. 2a ). Concordance can be further separated into SNPs and indels, with 79% and 57% overlapping, respectively (Supplementary Fig. 4 ). Variant overlap was further investigated to reveal its association with mutation caller, sample, and cancer type (Fig. 2a–c ). Consensus variant calling showed 91,705 (45.3%) concordant variants were captured in the intersection of Sanger, MuSE, DKFZ, and Broad callers from PCAWG, as well as Varscan, SomaticSniper, Radia, MuTect, and MuSE callers from MC3. Notably, an additional 7.7% were identified by all SNV mutation detection algorithms, except SomaticSniper. The reduced sensitivity of SomaticSniper is related to its algorithmic consideration of tumor contamination in the matched normal (e.g., skin) for liquid tumors [8] . After optimizing for filtering strategies, we performed a sample level comparison and found that 70% of samples had greater than 80% mutation concordance across the two cohorts. An additional 20% of samples had greater than 80% mutation recoverability in one or the other technique (Fig. 2b ). Skin Cutaneous Melanoma performed the best among all cancer types and had the highest variant-matching rates for both MC3 and PCAWG (Fig. 2c ). Generally, when considering all MC3 and all PCAWG mutations separately, we observed that PCAWG variant matching rates were generally higher, especially for Kidney Chromophobe (KICH), Brain Lower Grade Glioma (LGG), Ovarian Serous Cystadenocarcinoma (OV), Rectum Adenocarcinoma (READ), and Thyroid Carcinoma (THCA). The differences in OV are likely driven by whole genome amplified library preparation. Generally, the median fractions for matching MC3 variants were lower than those of matching PCAWG variants. This result was unexpected because MC3 provided fewer unique variants overall, suggesting that a large fraction of PCAWG unique variants reside in a few samples. Furthermore, after accounting for hypermutators, we identified a correlation between non-silent mutations per megabase and mean consensus percentages at the cancer level in both PCAWG consensus percentages (Mann–Whitney p -value = 1.97 × 10 −3 ) and MC3 consensus percentages (Mann–Whitney p -value = 6.59 × 10 −4 , see “Methods” section, Supplementary Fig. 1c, d ). Despite strong rank statistics, neither set exhibited strong correlation values for MC3 variants or PCAWG variants, R 2 statistics = 0.31 and 0.17 respectively with the majority of cancer types exceeding 80% mean concordance. Thus, one may expect to observe slightly higher variant fidelity in samples with more mutations. Fig. 2: Landscape of mutations overlap by caller, sample and cancer type. a UpSetR [41] plot shows the variant calling set intersection by caller. The y-axis indicates set intersection size and the x -axis uses a connected dot plot to indicate which sets are considered. Only the largest 27 intersecting sets are shown. Two insets of the UpSetR plot highlight a classic Euler diagram (left), which indicates the total number of overlapping mutations. A set-size bar chart (right) illustrates the total number of mutations considered from each caller. The concordance set indicates the agreement between WES and WGS. Indel callers are indicated with an asterisk. b A scatter plot shows the amount of concordance by sample by calculating the fraction of matched variants divided by the total number of mutations made by MC3 exome sequencing and PCAWG whole genome sequencing ( x and y -axis, respectively) below the total fraction of samples within each quadrant. Each point within the plot is related to tumor portion data collected from the TCGA barcode ID. c As shown above, this box plot separates panel b by cancer types (blue considers all MC3 variants, and red boxes indicate all PCAWG variants). Sample sizes are displayed for each cancer; points indicate samples that extend past 1.5 times the interquartile range; and horizontal bars within each box and whisker indicates median matched mutation fraction. Full size image Variant allele fraction affects call-rates After achieving a comparable data set and merging MC3 and PCAWG variants, we found that low VAF is the prevailing attribute of unique mutations. VAF is a fundamental factor in somatic variant detection, as well as sub-clonal structure prediction, and is used to predict subclonal tumor growth rates and metastatic potential. To explore the contribution of VAF, we sought to distinguish the contribution of subclonal structure and statistical chance when exploring private mutations in a single call set. We articulate our findings in six broad categories: modeling sequence noise, departure from idealized behavior, sub-clonal modeling, annotation differences, variant-caller effects, and analysis correlations. Association of variant allele fraction with recoverability We have observed that variants with low VAF are less likely to be reported in both call-sets. This finding relates to the lower sensitivity of somatic variant callers for variants with low VAF. To illustrate this principle, we estimated the expected overlap rate between MC3 and PCAWG at different VAFs. The sensitivity of MuSE across a range of VAFs and read depths in synthetic data was reported in Fan et al., 2016 [3] . We used these reported benchmarking characteristics of MuSE to estimate the expected overlap rate between the MuSE call-sets of MC3 and PCAWG across a range of VAFs (see “Methods” section). These expectations, which involve lower overlap rates at lower VAFs, generally tracked observed data but tended to overestimate observed overlap rates, especially for predicting the recovery fraction of MC3 variants in PCAWG. (Fig. 3a ) The discrepancies between expectations and observations may relate to simplifying assumptions that made this modeling possible (see “Methods” section). Fig. 3: Recoverability simulation and effects of subclones on mutation concordance. a Observed recovery rate of PCAWG variants in MC3 (red) and of MC3 variants in PCAWG (blue), alongside sequencing noise simulations calculated from random draws of a binomial model that incorporates the VAF and estimated read depth at each site (light red simulates PCAWG recoverability of MC3 variants, and light blue simulated MC3 recoverability of PCAWG variants). Y -axis is described with legend. X -axis displays VAF of the comparative data set in regard to Y . b A stacked bar chart displays the proportion of matched and unique variants ( y -axis) for different VAF bins ( x -axis). 180 variants did not provide read count information and were removed from this figure. c Stacked proportional histogram shows the fractions of PCAWG matched mutations (purple) and PCAWG-unique mutations (red). Mutations were restricted to SNVs, and subclonality predictions are indicated as either ‘Clonal’ or ‘Sub-clonal’. Columns 2–4 reflect sub-clonal assignment provided by PCAWG (Note: only a few samples reported five predicted subclones and were not included in this analysis). The number of variants represented for each clonal assignment is shown on the x -axis. d Similar to panel c , a stacked proportional histogram illustrates the proportion of matched and unique variants for MC3 which provide estimates of total number of matched or unique variants called by MC3. Full size image More generally, we observed that VAF had a greater association with variant recovery rates than predicted by the binomial model (Fig. 3b ). A random forest regression model trained on five statistics characteristics of VAF distribution per PCAWG sample and another five for that of the corresponding MC3 call-set predicted the fraction of variants per sample unique to PCAWG with 0.85 (0.86—when restricting to variants called by MuSE) Spearman correlation of test-set observations and a 0.68 (0.78) coefficient of determination (R 2 ). The strong association of VAF with recovery rates by call-set, despite modest explanatory power of the binomial, indicates important departures from idealized behavior. These departures could include explanations such as: PCR amplification violates the assumption of independence of reads, imputed read depths are systematically inflated, or some low-VAF variants represent sequencing artifacts. We conclude that non-ideal effects of VAF predict the majority of sample-level variance in fraction of co-called variants. Exploring subclonality One possible explanation for some variants being private to one call-set is that the sequencing aliquots for the two sequencing projects came from subclonally-distinct microregions of the same tumor. To investigate this possibility, we tested whether the MC3 and PCAWG call-sets differed from each other systematically at the subclonal level (Fig. 3c, d ). We hypothesized that tumors with a more complex subclonal structure (i.e., greater number of subclones) would have larger systematic differences in the VAF of shared variants between the MC3 and PCAWG call-sets. We found a small but highly significant effect: each additional subclone increased the average absolute difference in VAF of the shared variants between MC3 and PCAWG by 0.003, with a p -value of 1.3 × 10 −11 (linear regression); this effect reversed after controlling for tumor purity, indicating that the observed trend does not provide evidence of this interesting concept in re-sequencing (see “Methods” section for details). We do not have evidence that systematic VAF differences between call-sets of the same underlying sample associate with tumor heterogeneity. Real time effects of VAF differences between these two data sets can be observed using the online MAFit tool (Fig. 4 ). Fig. 4: Screenshots of online tool MAFit. Here we display screenshots from the MAFit on-line interface. Currently there are three main components to the interface: a A side panel shows sliders and radio buttons to filter data set to remain inclusive. In addition, a download button is available that will download the underlying data table. b MAFit rebuilds Fig. 2b in the first tab of the on-line interface. Each alteration to the radio buttons or VAF sliders will result in an updated figure. In addition, if one’s hovers over a point on the scatter plot, a pop-up window will automatically display, providing the user with basic statistics used to calculate that point, i.e., total number of mutations, number of unique and matched mutations. c A table is also presented based on the selection criteria in panel a . Full size image Annotation differs by call-set Genome annotation is critical for biological interpretation and downstream analysis of sequencing data. In order to avoid issues that arise from annotation differences, we only considered genomic locations in our intersection strategy. In doing so, we observed 2153 annotation differences where MC3 and PCAWG had different genes annotated for the same mutation. After restricting the mutation type to missense mutations and indels, 789 annotations differences remained. Most of these had the same mutation types annotated by both call-sets (690 SNPs, 15 insertions, 50 deletions), but some discrepancies remained. Notably, 413 out of 789 mismatch variants are labeled coding in MC3 but non-coding in PCAWG (Supplementary Data 4 ). We also observed four mutations that were annotated as cancer gene mutations by MC3, but as non-cancer gene mutations by PCAWG, and another four mutations that were annotated as cancer gene mutations by PCAWG, but as non-cancer gene mutations by MC3. One such example subsumed two mutations on chromosomal location 3p21.1 (genomic locations chr3:52442525 and chr3:52442604) that were annotated as missense mutations of BAP1 by MC3, but as 5’Flank SNPs of PHF7 by PCAWG. While identical pipelines resolve such differences, we stress the potential for misinterpretations when combining these publicly-available datasets. Effects of software Another important issue we assess is the degree to which differences in bioinformatics pipelines impact concordance. We extracted calls from MuSE and MuTect, both of which were executed on each dataset, and examined 6 subsets of results: MuSE-only-calls and all calls save MuSE-calls (the complement), MuTect-only-calls and their complement, and MuSE + MuTect calls and their complement. MuSE and Mutect each generate around 95% of the total calls, of which each respective subset shows close to 80% concordance between WES and WGS (Supplementary Fig. 5 ). These call sets themselves overlap almost completely, with their combination (MuSE + MuTect) giving a marginally higher concordance. Conversely, the data-specific caller combinations (referred to above as the complements) each furnish small call sets which vary considerably between WES and WGS (concordance as low as 15%). Because of the vast difference in the sizes of the MuSE/MuTect and the complementary call sets, there is little difference in the original analysis versus analyses restricted to variant callers common to both platforms. Differences in software pipelines do not appear to be significant confounding factors in concordance here. Effects on higher-level analysis We also sought to assess how higher-level analyses might be impacted using mutation signature analysis as a representative. We ran SignatureAnalyzer28 to ascertain signatures between matched WGS and WES samples for each case. A total of 563 of 739 cases (76%) showed the same dominant signature between WES and WGS and the multi-element signature vectors for each case are very highly correlated with one another, the average Pearson coefficient being almost 90%, with a cohort significance of <2 × 10 −6 (Fisher’s Test, “Methods” section, Supplementary Fig. 6 ). These observations suggest that signature analysis is relatively insensitive to data type when concordance is high, as it is here. Landscape of private WES and WGS mutations After identifying many possible sources of variation among private variants, we sought to characterize the fraction of variation explained by previously identified factors (Supplementary Fig. 7 , see “Methods” section). As displayed, subclonal and low VAF variants make up the largest fractions of explained variants for private MC3 and PCAWG variants. Notably, for private MC3 calls, indels (not called by MuSE or MuTect) are the next highest source of variation explained. GC-content and poor performing cancers such as THCA, KICH, and PRAD make up a smaller portion of the total number of private mutations. Variants present in only one public call-set We sought to classify cancer driver mutations uniquely identified by MC3. 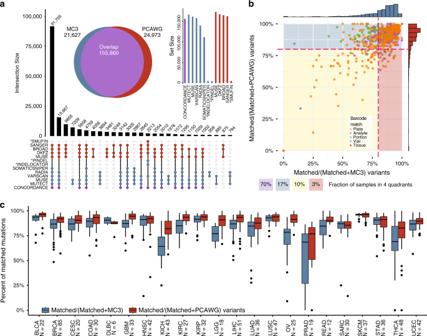Fig. 2: Landscape of mutations overlap by caller, sample and cancer type. aUpSetR41plot shows the variant calling set intersection by caller. The y-axis indicates set intersection size and thex-axis uses a connected dot plot to indicate which sets are considered. Only the largest 27 intersecting sets are shown. Two insets of the UpSetR plot highlight a classic Euler diagram (left), which indicates the total number of overlapping mutations. A set-size bar chart (right) illustrates the total number of mutations considered from each caller. The concordance set indicates the agreement between WES and WGS. Indel callers are indicated with an asterisk.bA scatter plot shows the amount of concordance by sample by calculating the fraction of matched variants divided by the total number of mutations made by MC3 exome sequencing and PCAWG whole genome sequencing (xandy-axis, respectively) below the total fraction of samples within each quadrant. Each point within the plot is related to tumor portion data collected from the TCGA barcode ID.cAs shown above, this box plot separates panel b by cancer types (blue considers all MC3 variants, and red boxes indicate all PCAWG variants). Sample sizes are displayed for each cancer; points indicate samples that extend past 1.5 times the interquartile range; and horizontal bars within each box and whisker indicates median matched mutation fraction. After removing two outlier samples having excesses of unique mutations (TCGA-CA-6717-01A-11D-1835-10, TCGA-BR-6452-01A-12D-1800-08), we observed 424 mutations in cancer genes [28] (median read depth = 97, median alternative allele count = 9) The four most frequently mutated genes were: KMT2C (22-mutations), PIK3CA (12), SPTA1 (9), and NCOR1 (9). Interestingly, the majority of unique PIK3CA mutations not identified by PCAWG were at 2 locations: E542K/G (5), and E545K (4). Whether this phenomenon reflects technical bias of WGS or is a product of subclonality warrants further investigation. The MC3 effort produced two mutation files: one controlled access somatic mutation file that represents nearly all mutations found by all callers, and a second was modified by the scientific community for public use. There are two critical differences in these files involving the reporting of mutations in exonic regions and mutations reported by a single variant caller. Since we limited our analysis strictly to exonic regions, we observed that 92% of the 9138 PCAWG private mutations found in the MC3 controlled access file were only identified by a single variant caller (Supplementary Fig. 8 ). As expected, the highest unique variant caller overlap was observed in MuTect and MuSE, two tools that were used by both MC3 and PCAWG. This observation accounts for 30% of PCAWG private variants. We investigated how many variants unique to the MC3 somatic public access call-set could be found in the PCAWG germline call-set for the same patients. We identified a total of six such variants (each in a different sample), five of which were flagged in the MC3 public call-set with one filter or another. Overall, this indicates that variants that have been incorrectly designated as germline or somatic are an extremely uncommon source of variation between the two projects. Variants in GC-extreme intervals Since it is well-known that the efficiency of exome capture is adversely affected by very high or very low GC-content [29] , [30] , we sought to test whether GC-content was associated with call rates in MC3 and PCAWG. We used a plug-in for VEP [31] to annotate all matched and private SNVs with CADD [32] in order to annotate each variant with the percentage of the neighboring 100 bases that are a G or C. First, we assessed how the distribution of read depth across GC-content changes between MC3 and PCAWG (Fig. 5b ). PCAWG was found to have a fairly uniform read depth across GC-content bins, while MC3 read depth was concentrated in regions of moderate GC-content (Fig. 5c ). The low read depth in MC3 at regions of extreme GC-content was in turn associated with lower variant recovery rates in these regions but did not grossly affect the number of variants recovered by MC3 because regions of extreme GC-content are relatively rare in the genome overall and in exome-capture regions in particular. Fig. 5: WGS mutations in exonic regions not captured by WES. a A sunburst diagram provides a breakdown of variants that are removed during the coverage step of the tool. The innermost circle represents the total number of variants identified upon filtering for exome beds used by MC3. Then, we restrict PCAWG variants to well-covered MC3 regions for each sample. The majority of gencode.v19 annotated and the BROAD target bed file of exonic regions are sufficiently covered by PCAWG in flanking regions: 3’UTRs, 5’UTR, and 5’Flanking. The outermost ring illustrates the number mutations identified by PCAWG that were poorly covered by MC3. b A density plot illustrates the density of percent GC-content from a 100 bp window surrounding a variant. Four variant-sets are displayed: matched, private to MC3, private to PCAWG, and we extend our dataset to include exonic variants not covered by WES but sufficiently covered in WGS (Covered by PCAWG only). c A scatter plot displays mean sequence depth ( y -axis) by increasing GC-content bins ( x -axis). Points are colored according to variant set (same as panel b ). d – f Total annotated mutations counts from 3 different annotated regions are shown for 5UTR, 3UTR, and missense mutations, respectively. g Expression Z −Scores for 3’UTR using all TCGA-UCEC samples. Cis -RNAseq expression violin plots are displayed for 13 genes. On top of the gene-level distribution violin plot, box and whisker plots display sample expression based on mutation classification (box include 25th quantile to 75th quantiles, and whiskers extend to 1.5 times the interquartile range). Full size image An in-depth analysis of these regions revealed that 76 mutations in known driver genes, identified in the combined TCGA data by Bailey et al. 2018, were missed in GC poor (GC fraction < 0.3) or GC rich (GC > 0.7) regions [28] . Three such instances revealed VHL mutations in KIRC that were overlooked in GC rich regions of this gene (two of these three recur). In addition, these 3 samples are not reported to carry a VHL mutation in the MC3 public data set. Other such instances include 7 SOX17 mutations, LATS2 (6), and CACNA1A (6). These findings emphasize the advantages of uniform coverage using WGS. The bases flanking a mutation (tri-nucleotide context) affect mutation rate, which should be approximately equal between MC3 and PCAWG, and also the rate of introduction of sequencing artifacts. Large differences in the call-rates of MC3 and PCAWG and particular nucleotide sequences could indicate a sequencing artifact unique to one or the other call-set, which might arise from different procedures for computationally filtering or biochemically preventing sequencing oxidation products. Therefore, we sought to test whether the trinucleotide context of variants correlated with relative call-rates in MC3 and PCAWG. Before applying the MC3 OxoG filters, we found a huge predominance of CA variants unique to MC3, with the trinucleotide contexts most specific to one database or another being 7-9 times more specific than the least specific trinucleotide contexts. After applying the MC3 OxoG filters, nucleotide contexts differed by less than four-fold in their specificities. The residual differential specificity by trinucleotide context after filtering can either indicate differences in sequencing artifact abundance and filtration by project, or could merely be a consequence of the fact that nucleotide context is also correlated with VAF and the distance from transcription start sites, which may independently affect MC3 and PCAWG relative call-rates. We extended the nucleotide context and performed mutation spectrum analysis, comparing all MC3 and all PCAWG mutations found after restricting the two data sets to exonic regions as described above (Step 3 of Fig. 1a ). We then calculated transition and transversion frequencies in each cancer type. After removing hypermutated samples and OxoG artifacts, we used a chi-squared test to determine the similarities and differences between cancer types in the full exome space compared versus the captured exome space. Strikingly, we did not identify significant differences in mutation spectrum in the majority of cancers. We did observe significant differences (FDR < 0.05) in the mutation spectrum for COAD, KICH, LUAD, and OV (Supplementary Data 5 ). These observations included strong discrepancies for AG and CG transition differences in KICH and OV, respectively. AT and CA transversions contributed mostly to COAD and LUAD differences (Supplementary Fig. 9 ). While these differences may reflect sequencing artifacts, such as whole genome amplified DNA in OV or low sample size, we believe the data can still provide more information pertaining to additional cancer genes and oncogenic mechanisms. Non-Coding/Flanking intersections with low coverage With the growing use of WGS in many labs, we sought to identify which mutations are gained by extending to this form of data. One major observation from our pipeline highlighted that some variants in exome regions were not well covered by WES (Fig. 1a Step 3). Using this mutation set we investigated the most recurrent members as derived by WGS but not by MC3 in exonic regions as defined by gencode.v19 (Fig. 5a ). We observed 697 mutations in cancer genes [28] uniquely called by WGS (Supplementary Data 6 ). We defined flanking mutations as all non-translated mutations near exons, i.e., 5’UTR, 3’UTR, 5’Flanking, and 3’Flanking regions, as they make up the majority of mutations not present in the MC3 public MAF. Recurrent mutation analysis identified the most frequently mutated genes in 5’UTR (Fig. 5d ), 3’UTR (Fig. 5e ), and missense mutations (Fig. 5f ). We found the most frequently mutated 3’UTR in cancer genes was PGR (91 mutations allowing for multiple mutations per sample), followed by ERBB4 (72), EPHA3 (42), CYLD (41), and PTPRD (34). To extend this analysis, we used RNAseq data collected by TCGA to determine mutation type specific cis- expression patterns, which clearly shows correlation of UTR mutations on RNA abundance (Fig. 5g ). Finally, similar to previous studies [33] , [34] , we investigated the potential effect of non-coding mutations when determining significantly mutated genes (SMG). Using MuSiC [35] with the no-skip-non-coding option, we rescued non-coding mutations annotated by PCAWG and included them in the significantly mutated gene (SMG) analysis. We only performed SMG analysis on cancer types having greater than 35 samples (BRCA-Breast-AdenoCa, HNSC-Head-SCC, KICH-Kidney-ChRCC, LIHC-Liver-HCC, LUAD-Lung-AdenoCA, LUSC-Lung-SCC, SKCM-Skin-Melanoma, STAD-Stomach-AdenoCA, THCA-Thy-AdenoCA, and UCEC-Uterus-AdenoCA). We initially identified potential driver-gene candidates ( FUT9 , MMP16 , SNHG14 , and SFTPB , Fig. 6 ) not previously reported in Pan-Cancer whole genome analysis, but further investigation did not support these candidates with the exception of SFTPB . Fig. 6: Significantly mutated gene analysis with the inclusion of UTR mutations. OncoPrint plots were generated using the R package ComplexHeatmap [42] for four cancer types: LUAD ( a ), LIHC ( b ), LUSC ( c ), and SKCM ( d ). We report all SMGs identified by Bailey et al. 2018 [28] , as well as top significantly mutated gene hits from MuSiC that include non-coding mutations. While many non-coding mutations look promising, further investigation yielded little support for driver identification status. Full size image SFTPB (FDR 1.56e−07) in LUAD was recently reported to be significantly mutated using a larger set of these same data [34] . As reported, this gene is involved in a lineage-defining surfactant protein. While six mutations contributed to its SMG status, only 1 3’UTR mutation was reported for LUAD in the MC3 controlled data set. Furthermore, this single indel was only found by one variant caller (Varscan). We confirmed the impact of SFTPB UTR mutations by performing a genome-wide association analysis of expression differences and found that samples with SFTPB mutations showed lower RNA abundance in PCDHA7 , a gene known to be involved in cells’ self-recognition and non-self-discrimination (chi-squared p -value 3.6 × 10 -8 ). While other promising candidates exist, such as FUT9 , a fucosyltransferase involved in organ bud progression during embryogenesis and has been implicated in cancer initiation [36] , we found no additional evidence for supporting its driver status. The research community is increasingly leveraging technology advances to integrate data at larger scales. We performed a comparative evaluation of ~750 samples with joint exome and whole genome sequencing mutation calls provided by two consensus mutation calling efforts, MC3 and PCAWG. This joint data set is encouraging, suggesting that ~80% of the predicted somatic mutations were captured by both efforts. Furthermore, a combined 90% of samples have greater than 80% variant concordance when considering covered exonic mutations from individual cohorts separately. Analysis of this data set also revealed three major contributors to variant discrepancies: (1) low variant allele fraction, (2) variant filtering decisions, and (3) technological limitations. Software differences were not an appreciable confounder. Distinct advantages and disadvantages accompany somatic mutation calling when utilizing captured WES or WGS. We found that ~70% of the discrepancies between whole genome and whole exome sequencing are influenced by low variant allele fraction. This information holds many implications in identifying subclonal heterogeneity in the tumor of interest. Other discrepant calls originate from the decisions made on how to filter and distribute publicly available mutation calls. Higher-order mutation signature analysis does not appear to be inordinately affected by these differences. We show that reported germline variants were negligible, but nearly 30% of the private PCAWG mutations were not reported by MC3 because only a single variant detection algorithm identified them. We want to emphasize that, while somatic variant detection in cancer is commonplace, there are still many issues to reconcile. Finally, we found additional mutations only observable in exonic regions using either WES or WGS. For example, WES uniquely identified 424 mutations in cancer genes with median VAF of ~10%. We also highlight ~700 WGS mutations from cancer genes, of which ~10% are attributable to regions of high and low CG-content; thus, highlighting the advantages of more uniform coverage from WGS. 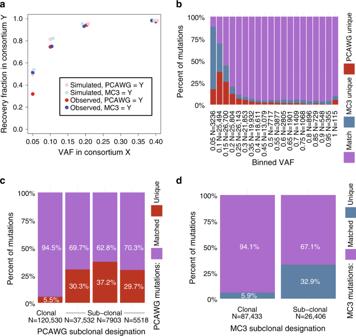Fig. 3: Recoverability simulation and effects of subclones on mutation concordance. aObserved recovery rate of PCAWG variants in MC3 (red) and of MC3 variants in PCAWG (blue), alongside sequencing noise simulations calculated from random draws of a binomial model that incorporates the VAF and estimated read depth at each site (light red simulates PCAWG recoverability of MC3 variants, and light blue simulated MC3 recoverability of PCAWG variants).Y-axis is described with legend.X-axis displays VAF of the comparative data set in regard toY.bA stacked bar chart displays the proportion of matched and unique variants (y-axis) for different VAF bins (x-axis). 180 variants did not provide read count information and were removed from this figure.cStacked proportional histogram shows the fractions of PCAWG matched mutations (purple) and PCAWG-unique mutations (red). Mutations were restricted to SNVs, and subclonality predictions are indicated as either ‘Clonal’ or ‘Sub-clonal’. Columns 2–4 reflect sub-clonal assignment provided by PCAWG (Note: only a few samples reported five predicted subclones and were not included in this analysis). The number of variants represented for each clonal assignment is shown on thex-axis.dSimilar to panelc, a stacked proportional histogram illustrates the proportion of matched and unique variants for MC3 which provide estimates of total number of matched or unique variants called by MC3. Only about 2% of the genome is protein coding. For the last dozen years, cancer genomics has provided a comprehensive molecular characterization of many different tumor types, thanks in large part to The Cancer Genome Atlas and other publicly funded efforts. The community is just starting to explore how exomics, transcriptomics, proteomics, and methylomics can be woven together across this 2% of the genome. We anticipate a general transition from WES to WGS, but this analysis is meanwhile reassuring that few clerical mutations were overlooked in WES and that WGS is capable of recapitulating previous genomic findings. Human research participants The Cancer Genome Atlas (TCGA) collected both tumor and non-tumor biospecimens from human samples with informed consent under authorization of local institutional review boards ( https://cancergenome.nih.gov/abouttcga/policies/informedconsent ). Sample overlap TCGA barcodes carry metadata that reflect tumor portions and different aliquots. As noted in Fig. 1b , TCGA barcode differ slightly in the comparison between MC3 and WGS aliquots. A brief description of the breakdown of the TCGA barcode is outlined below. Example: TCGA-DD-0001-01B-01D-A152 - TCGA-Project - DD-Tissue source site: the tissue location of tumor that matches clinical metadata. - 0001-Participant code - 01-Sample type: i.e., solid tumor (01), primary blood derived tumor (03), solid tissue normal (11), blood derived normal (10) - B-Vial: the order in a sequence of samples, i.e., A = first in sequence, B = second in sequence - 01-Portion: sequential order of the 100–120 mg of samples - D-Analyte: molecular analyte type for analysis, i.e., D for DNA and W for WGA. - A152-Plate: sequential location of a 96-well plate A lookup table outlining these fields is located at the GDC: https://gdc.cancer.gov/resources-tcga-users/tcga-code-tables . In order to determine the role of aliquot differences in assessing mutation concordance, we re-analyzed the clonality and overall mutation overlap after stratifying for exact barcode differences. We observed that the effect of matching barcodes on match variant frequency has little effect. Assessing cancer subtype selection preference Analysis working groups for TCGA projects were primarily subdivided according to cancer types. Scientific experts gathered in consortia from around the country to participate in characterizing many tumors using high throughput data generated on many substrates, e.g., WES, RNAseq, etc. At the conclusion of these projects, groups were asked to hand-select a subset of samples to perform validation sequencing (WGS, the samples used in this analysis). The selection criteria differed from group-to-group and sometimes resulted in an overabundance of one subtype over another. To determine cancer subtype selection bias, we performed an enrichment analysis. Using clinical data we calculated (for each cancer type) the subtype fraction in the WES cancer cohort and measured whether the fraction was similar to WGS set of samples using a Fisher’s exact test. Defining exonic regions We used the same definition as Ellrott et al. to reduce whole genome and exome calls to define genomic coordinates [27] . Coverage calculations Fixed-step (step = 1) Wiggle coverage files (.wig) for both MC3 and PCAWG were provided by the Broad Institute. The wig format is a binary readout of sufficient sequencing coverage for genomic data. Here, sufficient coverage is defined as bases with 8 or more reads at a given location. These wig files were processed and reduced to exonic regions using the wig2bed function from BEDOPTS [37] . After the preliminary screen of coverage-reduced MAF files, we observed that matching mutations (identified by PCAWG and MC3) were removed from one technology and not the other after the coverage reduction step. To account for this issue, we performed a self-coverage reduction step to that identified 6460 mutations. We describe some properties of those mutations here. The median tumor depth reported by MC3 from these variants is 12 reads (+/− 3 median absolute difference). The median tumor depth reported by PCAWG in this region is 39 reads (+/− 35.6 median absolute difference), suggesting wide variance of tumor read depths that were removed. However, the mode tumor depth of the PCAWG variants was 13, justifying this removal of variants with low read support. Finally, we determined how many of these poorly-covered variants originated from cancer driver genes. We observed 126 mutations from the MC3 file, and 156 cancer mutations were eliminated at this stage in the comparison. Overlapping mutations After reducing the variants to be within exome sequencing target region, within same exon definitions, and having enough sequencing depth, the remaining variants from ICGC and PCAWG were stored in a SQLite database to enable fast lookup. We then executed a full join between the two sources of variants by matching the donor ID, sample ID, and the genomic range of each variant. The full join output was further cleaned up to remove duplicated filters due to naming variations and duplicated variants due to DNPs. - Matching IDs - Matching chromosomes - End position greater than or equal to start position - Start position is less than or equal to end position. Deduplication of variants After merging the PCAWG and MC3 data, we observed different strategies were taken by MC3 and PCAWG to capture neighboring variants, i.e., complex indels, di-nucleotide (DNP) and tri-nucleotide (TNP) polymorphisms. To address complex indel events (SNVs in indel regions), the MC3 working group absorbed the variants made by SNV callers into the assignment made by Pindel. Conversely, PCAWG merged DNP and TNP events into a single event. These strategies resulted in many duplication events from MC3 and PCAWG: 1731 and 62, respectively. These events encompassed 3457 and 119 events, respectively. To address these differences, we merged PCAWG variants into MC3s complex indel events, and MC3 variants into single DNP or TNP events. Filtering optimization After reducing the starting pool of possible mutations from 746 samples to covered exons, we sought to identify the optimal set of MC3 filters that provide the largest number of samples with greater than 80% concordance from the two technologies with the simplest schema. This was performed comprehensively using all possible combinations of filters, often with more than one filter per variant, with the MC3 cohort (131,071 filter combinations). Filter flags include: “common_in_exac”, “gapfiller”, “native_wga_mix”, “nonpreferredpair”, “oxog”, “StrandBias”, and “wga”. We pre-defined the exclusion of variants in MC3 flagged as OxoG along with the inclusion of all PASS variants. The comprehensive filter analysis resulted in two major clusters of variant recoverability (Supplementary Fig. 3 ). Here, we observed the computational trade-off of identifying more matched variants at the cost of more unique MC3 calls. Below, we highlight five strategies considered for analysis (Supplementary Data 2 ). 1. Only consider variants labeled PASS by the MC3 filter column. 2. Only remove variants labeled OxoG by MC3. 3. Prioritize G1 (samples in the most recoverable quadrant, MC3 and PCAWG samples with greater than or equal to 80% from both efforts.) 4. Prioritize total number of matched variants. 5. Maximize total number of samples in the most recoverable quadrant (Fig. 2b ) while maximizing the difference between unique MC3 variants and matched variants thus generating fewer unique calls. After considering complexity, we chose to move forward with strategy 2 for the entirety of this study due to its simplicity and relative similarity to other filtering schemes. We recognize that by selecting a single filtering strategy, we are limiting the data slightly and likely introducing some false positive variant calls. However, this strategy allowed us to maintain larger sample sizes and to capture ~15,000 more matched variants than the PASS only strategy at the cost of ~3500 unique mutations calls for MC3. Assessing mutations per megabase and cancer type concordance Mutations per megabase data were collected from the broader TCGA dataset and reduced following the same methods outlined previously [28] . Briefly, this systematically removed hypermutators from the dataset. This resulted in a set of 625 samples from the MC3/PCAWG dataset studied here and 8852 TCGA samples. Both Pearson and Mann-Whitney correlations statistics were performed to assess the association of non-silent mutations per megabase and concordance statistics. Simulation of sequencing noise and recoverability Fan et al. benchmarked the sensitivity of MuSE at recovering somatic variants across 24 combinations of VAF and read depth [3] . When simulating the recovery of PCAWG variants in MC3 we assumed that the VAF observed in PCAWG was the true VAF. We matched the observed VAF of each variant to the closest VAF reported in Fan et al. 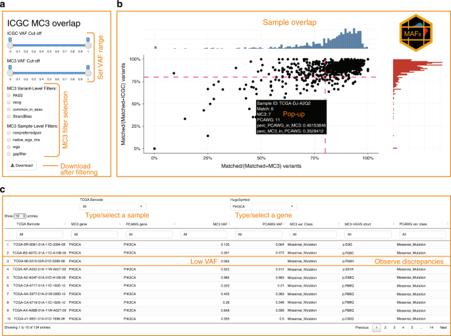Fig. 4: Screenshots of online tool MAFit. Here we display screenshots from the MAFit on-line interface. Currently there are three main components to the interface:aA side panel shows sliders and radio buttons to filter data set to remain inclusive. In addition, a download button is available that will download the underlying data table.bMAFit rebuilds Fig.2bin the first tab of the on-line interface. Each alteration to the radio buttons or VAF sliders will result in an updated figure. In addition, if one’s hovers over a point on the scatter plot, a pop-up window will automatically display, providing the user with basic statistics used to calculate that point, i.e., total number of mutations, number of unique and matched mutations.cA table is also presented based on the selection criteria in panela. For our analysis, the best value to use as the read depth when predicting the MC3 recovery rate of PCAWG variants would be the MC3 read depth at the same site and sample as the PCAWG variant. However, it was not practical to obtain MC3 read depths at sites without MC3 variants, so instead we simulated an MC3 read depth for each PCAWG variant by randomly sampling from the read depths of observed MC3 variants from the same sample as the PCAWG sample. We then matched these simulated read depths for each variant to the closest read depths reported in Fan et al. For the binned VAFs and read depths for each PCAWG variant obtained as above, we pulled the corresponding sensitivities of MuSE from the Fan et al. paper and simulated MC3 variants with probability equal to these sensitivities. Integrating clonality Both consortia considered clonality in their comprehensive characterization of the somatic mutations. 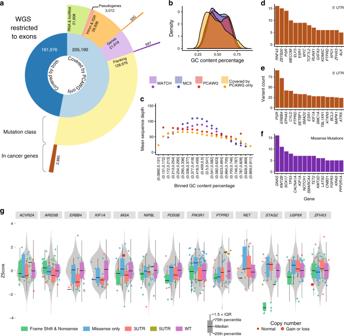Fig. 5: WGS mutations in exonic regions not captured by WES. aA sunburst diagram provides a breakdown of variants that are removed during the coverage step of the tool. The innermost circle represents the total number of variants identified upon filtering for exome beds used by MC3. Then, we restrict PCAWG variants to well-covered MC3 regions for each sample. The majority of gencode.v19 annotated and the BROAD target bed file of exonic regions are sufficiently covered by PCAWG in flanking regions: 3’UTRs, 5’UTR, and 5’Flanking. The outermost ring illustrates the number mutations identified by PCAWG that were poorly covered by MC3.bA density plot illustrates the density of percent GC-content from a 100 bp window surrounding a variant. Four variant-sets are displayed: matched, private to MC3, private to PCAWG, and we extend our dataset to include exonic variants not covered by WES but sufficiently covered in WGS (Covered by PCAWG only).cA scatter plot displays mean sequence depth (y-axis) by increasing GC-content bins (x-axis). Points are colored according to variant set (same as panelb).d–fTotal annotated mutations counts from 3 different annotated regions are shown for 5UTR, 3UTR, and missense mutations, respectively.gExpressionZ−Scores for 3’UTR using all TCGA-UCEC samples.Cis-RNAseq expression violin plots are displayed for 13 genes. On top of the gene-level distribution violin plot, box and whisker plots display sample expression based on mutation classification (box include 25th quantile to 75th quantiles, and whiskers extend to 1.5 times the interquartile range). 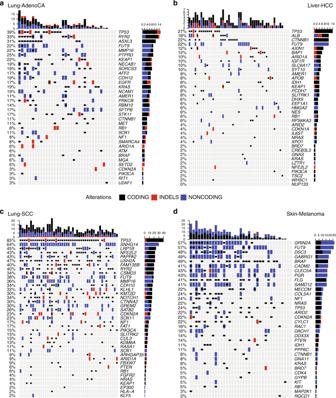Fig. 6: Significantly mutated gene analysis with the inclusion of UTR mutations. OncoPrint plots were generated using the R package ComplexHeatmap42for four cancer types: LUAD (a), LIHC (b), LUSC (c), and SKCM (d). We report all SMGs identified by Bailey et al. 201828, as well as top significantly mutated gene hits from MuSiC that include non-coding mutations. While many non-coding mutations look promising, further investigation yielded little support for driver identification status. Locations of these files are provided in the data availability section. Here, we provide a brief summary of the strategies used to compile these resources. First, the PanCancer Atlas working-groups used MC3 mutations to predict subclonal structures using ABSOLUTE [38] . This tool uses copy number, recurrent karyotype, and mutation data to calculate copy number purity and cluster identification. Furthermore, the PanCancer Atlas working group only made the distinction of clonal and subclonal mutations and did not attempt to further assign sub-clonal mutations to other likely heterogeneous clusters. PCAWG, on the other hand, used a consensus calling approach incorporating 11 different clustering tools. Here, we evaluated cluster-ID which represents those mutations that are clonal (ID = 1), with other clusters representing mutations that are subclonal (ID = 2 through 4). For this analysis, we restricted our data to SNVs to be consistent with calls made by the PanCancer Atlas calls of MC3 mutations. Fraction of private variation explained In Supplementary Fig. 7 we provide a breakdown of different sources of variant described in our analysis using publicly available data. For MC3 all private variants were classified as into 3 variant types (Indel, MissensePlus, and Other). Specifically, indels are comprised of: “Frame_Shift_Del”, “In_Frame_Ins”, “Frame_Shift_Ins”, and “In_Frame_Del”. MissensePlus variants are comprised of: “Missense_Mutation”, “Nonsense_Mutation”, “Nonstop_Mutation”, “Splice_Site”. And Other variants are comprised of: “RNA”, “3’UTR”, “5’UTR”, “5’Flank”, “Silent”, “3’Flank”, “Intron”, “Translation_Start_Site”. On the other hand, PCAWG variants were also categorized into Indels, MissensePlus, and Other. Specifically, indels are comprised of: “Frame_Shift_Del”, “Frame_Shift_Ins”, “De_novo_Start_InFrame”, “Start_Codon_Ins”, “Stop_Codon_Ins”, “In_Frame_Del”, “In_Frame_Ins”, “Stop_Codon_Del”, and “Start_Codon_Del”. MissensePlus variants are comprised of: “Missense_Mutation”, “Nonsense_Mutation”, “Nonstop_Mutation”, “Splice_Site”. And other variants are comprised of: “5’UTR”, “RNA”, “5’Flank”, “Silent”, “3’UTR”, “Intron”, “IGR”, “lincRNA”, “De_novo_Start_OutOfFrame”, and “Start_Codon_SNP”. In addition to the three variant type categories, six additional sources of variation were added to private variants: Subclonal, VAF5, VAF10, MMcomplement, THCA KICH or PRAD, and GCcontents. As mentioned, subclonal variants are tagged if labeled as identified by the TCGA or ICGC consortia. VAF5 tags all variants with less that 5% VAF. VAF10 tags all variants with VAF greater than or equal to 5% and less that 10%. MMcompelement tags all variants not detected by MuSE or MuTect. And finally, GCcontent was calculated as the fraction of G or C nucleotides in a 100 bp window surround a variant. This was calculated using a CADD plug-in to VEP. The GCcontent flag was assigned to a variant if GC fraction was less and 0.3 or greater than 0.7. MAFit: online comparison and visualization tool MAFit (maf Interaction Tool) is a shinyapp [39] tool to visualize and extract mutations from the intersection of PCAWG and MC3 call sets. It is an interactive and graphical web-based interface built using R Shiny. The interface consists of three panels: a main scatter plot display, a side box of control widgets, and a mutation table in the bottom pane. Any alteration of a control widget will update the scatter plot and the mutation table, enabling very rapid browsing. There is also a button to download the current data set displayed in the scatter plot. The main panel displays a scatter plot with marginal histograms of mutations grouped by sample. The axes are percentage of matched mutations versus matched plus call-set-unique mutations. Mouse-hovering on a data point initiates a pop-up window showing specific information for this sample, such as TCGA barcode, number of matched mutations, and numbers of mutations unique to each call-set. The side panel contains two sets of control widgets which can be used to select data based on different criteria. The top control set consists of two sliders to set the VAF cut-offs for each call-set. Both ends of the slider can be adjusted so that users can obtain a desired interval of the VAF. The bottom control set consists of check-boxes of both variant-level and sample-level MC3 filters. If only variant-level filters are checked, all PCAWG-only mutations will be retained; if at least one sample-level filter is checked, mutations from samples that do not have any checked filters flagged (variant-level or sample-level) will be filtered out. Both variant-level and sample-level filters result in the union of mutations with any checked filter will be shown. The bottom panel displays a table of mutations based on the selection criteria from the side panel. Columns include information on each mutation, such as TCGA barcode, gene name, VAF, variant class, Human Genome Variant Society (HGVS) nomenclature, etc. Users can sort the table by each column. There are two drop-down selection boxes where users can view mutations from a specific TCGA barcode or Hugo symbol. There is also a search bar, which results in mutations that contain the input in any columns. Controlled access files Having worked with both the TCGA and ICGC consortia, we were privy to the controlled access data (all MC3 somatic variant calls and PCAWG germline calls). These data sets allowed for the further interrogation of unique variants called by both groups. We performed a mutation variant intersection of MC3 controlled access mutations with unique PCAWG variants in the captured exonic regions. These data can be downloaded using necessary credentials from https://gdc.cancer.gov/about-data/publications/mc3-2017 . We intersected the MC3 public MAF with the PCAWG germline call-set, donor-by-donor. Six MC3 somatic variants were identified as germline variants in PCAWG for the same donor. Of these, five were flagged in MC3 as OxoG or non-preferred-pair artifacts, and only one was marked PASS in MC3. This PASS variant had a depth in the matched MC3 normal of well over 100 with no alternate reads. The minimal intersection between the MC3 somatic call-set and the donor-matched PCAWG germline call-set is evidence that germline contamination in MC3 calls is low. Assessment of impact on mutation signature analysis We ran SignatureAnalyzer [40] on the corpus of WES and WGS samples from our TCGA cases. This tool reports a vector of J = 7 normalized weights corresponding to mutational signatures. Once weights were computed, we used COSMIC signatures as a reference in order to synchronize labels of the fractional weights between WES and WGS data for each case to enable proper comparison. We excluded 5 cases in which signatures were not computed for WGS data. Using the synchronized results, we then assessed both the number of cases for which the tool identified the same dominant signature between WES and WGS data and also evaluated the correlation between WES and WGS vectors for each case using least-squares regression. Statistical significance of each correlation was calculated using a 2-tailed t -test. Statistical power of each correlation was limited by the paucity of signature weights because the underlying t-statistic is proportional to the square root of J – 2. However, because these cases, and therefore their hypothesis tests, are independent, the cohort constitutes multiple tests of the same hypothesis regarding signatures derived from WES and WGS data. Therefore, we combined individual P-values into an overall cohort P -value using Fisher’s log-transform. Namely, the transform of negative 2 times the natural log of the product of the K = 739 individual P -values is, itself, chi-square distributed with 2 K degrees of freedom. Using this transform, we found an overall cohort P -value of <2 × 10 −6 . Reporting summary Further information on research design is available in the Nature Research Reporting Summary linked to this article.